Impaired mitochondrial oxidative metabolism in skeletal progenitor cells leads to musculoskeletal disintegration Although skeletal progenitors provide a reservoir for bone-forming osteoblasts, the major energy source for their osteogenesis remains unclear. Here, we demonstrate a requirement for mitochondrial oxidative phosphorylation in the osteogenic commitment and differentiation of skeletal progenitors. Deletion of Evolutionarily Conserved Signaling Intermediate in Toll pathways (ECSIT) in skeletal progenitors hinders bone formation and regeneration, resulting in skeletal deformity, defects in the bone marrow niche and spontaneous fractures followed by persistent nonunion. Upon skeletal fracture, Ecsit-deficient skeletal progenitors migrate to adjacent skeletal muscle causing muscle atrophy. These phenotypes are intrinsic to ECSIT function in skeletal progenitors, as little skeletal abnormalities were observed in mice lacking Ecsit in committed osteoprogenitors or mature osteoblasts. Mechanistically, Ecsit deletion in skeletal progenitors impairs mitochondrial complex assembly and mitochondrial oxidative phosphorylation and elevates glycolysis. ECSIT-associated skeletal phenotypes were reversed by in vivo reconstitution with wild-type ECSIT expression, but not a mutant displaying defective mitochondrial localization. Collectively, these findings identify mitochondrial oxidative phosphorylation as the prominent energy-driving force for osteogenesis of skeletal progenitors, governing musculoskeletal integrity. Mitochondrial diseases are associated with decreased energy production in organs with high energy requirements and are mainly due to defects in the oxidative phosphorylation (OXPHOS) machinery [1] , [2] , [3] , [4] . Releasing energy through OXPHOS requires the orchestrated action of five multi-heteromeric enzyme complexes (complexes I–V), located in the inner mitochondrial membrane [5] . Mitochondrial complex 1 (CI) is the largest complex comprised of at least 45 different proteins and is the primary entry point that generates the proton motive force for electrons into the electron transport chain driving ATP production [6] , [7] , [8] . CI-deficiency is the most frequent cause of defects of the OXPHOS system that cause multisystem dysfunction [9] , [10] , [11] , [12] , [13] , including skeletal disorders [14] , [15] . Emerging epidemiological evidence [16] , [17] , [18] and data from animal models [3] , [19] suggest an association of mitochondrial dysfunction and high oxidative stress with skeletal disorders, including a clinically significant decrease in bone strength, reduced bone mineral density, premature aging of bone or a high risk or fragility fractures. For example, Kearns Sayre Syndrome (KSS), a rare mitochondrial DNA deletion syndrome, shows clinical manifestations of muscle weakness and wasting, accompanied with multiple bone deformities and severe fractures, causing loss of the ability to walk and early lethality [20] . In addition, mitochondrial respiratory chain deficiency is related to spontaneous bone fractures and myopathy [21] . However, it is unclear how mitochondrial defects contribute to skeletal dysfunction associated with myopathy. Glycolysis is the primary metabolic process that generates ATP for energy and intermediate metabolites, including active lipids, nucleotides, and amino acids, for biosynthesis [22] , [23] . It serves as the major energy and carbon source for committed osteoblast-lineage cells during osteogenic differentiation [22] , [24] , [25] , [26] . In particular, metabolic intermediates fuel the synthesis of amino acids to produce extracellular matrix proteins and hydroxyapatite in bone [22] . In addition to glycolysis, glutamine metabolism also provides osteoblast progenitors with an additional energy source as well as a carbon and nitrogen source [26] . Glutamine is converted to citrate through the tricarboxylic acid (TCA) cycle in the mitochondria, producing ATP through the OXPHOS pathway, while providing metabolic intermediates for the synthesis of amino acids, nucleotides, glutathione, and hexoamine [27] . Recent studies demonstrated an in vivo role for glutamine and glucose metabolism in skeletal progenitors using conditional deletion of the enzyme glutaminase (Gls) and the glucose transporter Glut1, respectively. Gls-deficiency in Prx1 + skeletal progenitors impaired,cell proliferation and osteogenesis during bone remodeling while Glut1-deficiency in Prx1 + skeletal progenitors abolished chondrogenesis, not osteogenesis, during skeletal development [28] . Notably, glutamine is likely to serve as major substrates for biosynthetic and antioxidant demands, not an energetic substrate, in skeletal progenitors since GLS inhibition did not induce any energetic alteration [29] . Thus, other energy metabolic pathways controlling osteogenesis of skeletal progenitors remain to be elucidated. To investigate in vivo roles for mitochondrial oxidative metabolism in musculoskeletal system, we developed a mouse model for mitochondrial CI deficiency by conditionally deleting Ecsit in multiple skeletal and muscle cells. Herein, we highlight the importance of mitochondrial OXPHOS in determining the osteogenic commitment and differentiation of skeletal progenitors as a critical rheostat of skeletal and muscular development. Notably, restoration of impaired OXPHOS pathway using recombinant adeno-associated virus (rAAV) may represent an untapped therapeutic avenue for mitochondrial disorders in the musculoskeletal system. Ecsit -deficiency in skeletal progenitors impairs early skeletal development The CI intermediate assembly (MCIA) complex, containing the core subunits (ECSIT, NDUFAF1, ACAD9, and TMEM126B) is required for the formation of mitochondrial complex I (CI) [6] , [30] , [31] , [32] , [33] . Among these subunits, ECSIT is highly expressed in skeletal cells, including endosteal osteoblasts, osteocytes, periosteal cells, and osteoclasts (Fig. 1a ), and its deficiency reduces the expression of other MCIA and CI components [31] , [32] , [33] . Mitochondrial localization of ECSIT in human bone marrow-derived stromal cells (BMSCs) and mouse osteoblasts residing on the surface of trabecular and cortical bones was also confirmed by immunofluorescence and subcellular fractionation analyses (Fig. 1b, c ). The role of mitochondrial activity in bone formation was examined in vivo using mice with targeted deletion of Ecsit in skeletal progenitors ( Ecsit Prx1 ). Deletion efficiency of Ecsit in these cells was confirmed by fluorescence microscopy and immunoblotting analyses (Supplemental Fig. 1a , Fig. 2c ). Ecsit Prx1 mice developed limb deformities along with spontaneous fractures in long bones right after birth (Fig. 1d , right). At postnatal day 21 (P21), they displayed severe osteoporosis and delayed formation of primary and secondary ossification centers in long bones (Fig. 1d, e , Supplemental Fig. 1b, c ). Severe hypomineralization and delayed formation of primary ossification centers was also evident in Ecsit Prx1 embryos and neonates (Fig. 1f , Supplemental Fig. 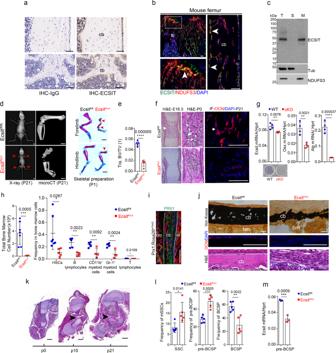Fig. 1:EcsitPrx1mice show defects in skeletogenesis, fracture healing, and the bone marrow niche. aImmunostaining of ECSIT in 2-month-old wild-type femurs. tb: trabecular bone, cb: cortical bone.bImmunofluorescence showing the localization of ECSIT in P21 mouse femurs. Arrows indicate co-localization of ECSIT and NDUFS3.c. Immunoblot analysis showing mitochondrial fractionation of ECSIT in human BMSCs.d,eX-radiography (d,left) and microCT showing P21 whole body and hindlimbs (d,middle) and quantification of femoral bone mass (e,n= 5). Alizarin red/alcian blue staining of P1 neonates (d,right). Arrows indicate spontaneous fractures. Tra. BV/TV: Trabecular bone volume/total volume.fH&E staining of E16.5 and P0 femurs (left,middle). Immunofluorescence showing osteocalcin (OCN) expression in the femurs (right). Arrows indicate femoral trabecular bone.gSkeletal progenitors isolated by FACS from P0Ecsit;Prx1Rosa26mTmG(cKO) andPrx1;Rosa26mTmG(WT) limbs using GFP+CD45−Ter119−Tie2−markers. Osteogenic gene expression (n= 4) and alkaline phosphatase activity (ALP,n= 3) were assessed for osteogenic differentiation.hFlow cytometry analysis showing frequency of the indicated bone marrow cell populations at P10 (right, HSCs (Ecsitfl/fl,n= 7;EcsitPrx1,n= 5); other subpopulations,n= 4−5) and total number of the isolated cells (left,Ecsitfl/fl,n= 7;EcsitPrx1,n= 6). Supplemental Fig.2demonstrates the gating strategy for this analysis.iGFP-expressing PRX1-lineage cells residing in the diaphyseal periosteum of P1PRX1-cre;Rosa26mTmGmice. m: muscle, bm: bone marrow.jP21 femoral cortical bones were stained for Von Kossa (top), H&E (bottom) and immunofluorescence for OCN (middle).kH&E staining ofEcsitPrx1femurs at the age of P0, P10, and P21.l,mFlow cytometry analysis showing frequency of SSCs, pre-BCSP, and BCSP in skeletal cells (l,n= 5). RT-PCR shows expression ofEcsitin pre-BCSP (m,n= 3). Supplemental Fig.3demonstrates the gating strategy for this analysis. A two-tailed unpaired Student’st-test for comparing two groups (e,g,h,l,m; error bars, data represent mean ± SD). Data are representative of three independent experiments. Scale bars =a, 100 μm;b, 50 μm;d (left, middle), 2 mm;d (right), 1 mm;f, 60 μm;i, 75 μm;j, 40 μm;k, 500 μm. 1e, f , Supplemental Table 1 ). Consistent with immunofluorescence analysis showing nearly complete absence of osteocalcin (OCN)-expressing mature osteoblasts in the femur of P21 Ecsit Prx1 mice (Fig. 1f , right), cKO Prx1 + skeletal progenitors, isolated from P0 Ecsit Prx1 hindlimbs as Prx1 + CD45 - TIE2 - TER119 - cells, failed to differentiate into mature osteoblasts (Fig. 1g ). Of note, the bone marrow niche function of Ecsit Prx1 skeletal cells was also disrupted, as shown by a significant reduction in total bone marrow cell numbers and a low frequency of hematopoietic stem cells (HSCs), B cells, macrophages, granulocytes, and T cells (Fig. 1h , Supplemental Fig. 2 ). These results suggest that ECSIT is essential for osteogenesis of Prx1 + skeletal progenitors and for the formation of bone marrow HSC niche. Notably, GLUT1-mediated glucose metabolism mediates chondrogenesis, not osteogenesis of Prx1 + skeletal progenitors [28] while GLS-mediated glutamine metabolism in Prx1 + skeletal progenitors is dispensable for skeletal development [29] . Thus, ECSIT-mediated mitochondrial regulation, not GLUT1-mediated glucose metabolism or GLS-mediated glutamine metabolism, plays a critical role in the osteogenic activity of Prx1 -lineage skeletal progenitors. Fig. 1: Ecsit Prx1 mice show defects in skeletogenesis, fracture healing, and the bone marrow niche. a Immunostaining of ECSIT in 2-month-old wild-type femurs. tb: trabecular bone, cb: cortical bone. b Immunofluorescence showing the localization of ECSIT in P21 mouse femurs. Arrows indicate co-localization of ECSIT and NDUFS3. c . Immunoblot analysis showing mitochondrial fractionation of ECSIT in human BMSCs. d , e X-radiography ( d , left ) and microCT showing P21 whole body and hindlimbs ( d , middle ) and quantification of femoral bone mass ( e , n = 5). Alizarin red/alcian blue staining of P1 neonates ( d , right ). Arrows indicate spontaneous fractures. Tra. BV/TV: Trabecular bone volume/total volume. f H&E staining of E16.5 and P0 femurs ( left , middle ). Immunofluorescence showing osteocalcin (OCN) expression in the femurs ( right ). Arrows indicate femoral trabecular bone. g Skeletal progenitors isolated by FACS from P0 Ecsit; Prx1 Rosa26 mTmG (cKO) and Prx1;Rosa26 mTmG (WT) limbs using GFP + CD45 − Ter119 − Tie2 − markers. Osteogenic gene expression ( n = 4) and alkaline phosphatase activity (ALP, n = 3) were assessed for osteogenic differentiation. h Flow cytometry analysis showing frequency of the indicated bone marrow cell populations at P10 ( right , HSCs ( Ecsit fl/fl , n = 7; Ecsit Prx1 , n = 5); other subpopulations, n = 4−5) and total number of the isolated cells ( left , Ecsit fl/fl , n = 7; Ecsit Prx1 , n = 6). Supplemental Fig. 2 demonstrates the gating strategy for this analysis. i GFP-expressing PRX1-lineage cells residing in the diaphyseal periosteum of P1 PRX1-cre;Rosa26 mTmG mice. m: muscle, bm: bone marrow. j P21 femoral cortical bones were stained for Von Kossa ( top ), H&E ( bottom ) and immunofluorescence for OCN ( middle ). k H&E staining of Ecsit Prx1 femurs at the age of P0, P10, and P21. l , m Flow cytometry analysis showing frequency of SSCs, pre-BCSP, and BCSP in skeletal cells ( l , n = 5). RT-PCR shows expression of Ecsit in pre-BCSP ( m , n = 3). Supplemental Fig. 3 demonstrates the gating strategy for this analysis. A two-tailed unpaired Student’s t -test for comparing two groups ( e , g , h , l , m ; error bars, data represent mean ± SD). Data are representative of three independent experiments. Scale bars = a , 100 μm; b , 50 μm; d (left, middle) , 2 mm; d (right) , 1 mm; f , 60 μm; i , 75 μm; j , 40 μm; k , 500 μm. Full size image Prx1-lineage skeletal cells are major cell populations (Fig. 1i ) that initiate callus formation and vascularization for successful bone fracture repair [34] , [35] , [36] . Ecsit deletion in Prx1 + skeletal progenitors resulted in nearly complete arrest of cortical bone and periosteal formation despite expansion of Ecist -deficient periosteal cells (Fig. 1j , Supplemental Fig. 1f ). Accordingly, Ecsit Prx1 femurs show spontaneous fractures occurring after birth. The resulting fracture sites displayed persistent nonunion with a lack of callus mineralization and mature osteoblasts and the persistence of an unmineralized fibrous callus with cartilaginous elements (Fig. 1j, k , Supplemental Fig. 1d ). To define where ECSIT is required in the osteoblast maturation process, skeletal cell populations were isolated from P0 Ecsit Prx1 limbs and subjected to flow cytometry [37] , demonstrating an increased frequency of skeletal stem cells (SSCs) and pre-bone, cartilage, stromal progenitors (pre-BCSPs) and a decreased frequency of BCSPs (Fig. 1l, m , Supplemental Fig. 3 ). Thus, Ecsit deletion in Prx1 + skeletal progenitors impairs the differentiation of SSCs and pre-BCSPs to BCSPs, resulting in defective commitment and differentiation of skeletal progenitors to osteoblasts. To test whether Ecsit deletion in skeletal progenitors is a primary cause of impaired fracturing healing in Ecsit Prx1 mice, Ecsit fl/fl mice were crossed with Prx1-Cre ERT2 -EG FP mice ( Ecsit Prx1-ERT/GFP ) to delete ECSIT expression in skeletal progenitors in an inducible manner. Fracture surgery was performed on the femurs of 6-week-old Ecsit Prx1-ERT/GFP and Prx1-ERT/GFP control mice three days after tamoxifen injection (Supplemental Fig. 4a ). One month later, tamoxifen-induced expression of Cre recombinase and deletion of Ecsit were validated by fluorescence microscopy and RT-PCR, respectively (Supplemental Fig. 4b, c ). MicroCT analysis revealed that basal bone mass in control and Ecsit Prx1-ERT/GFP femurs was comparable, as shown by equivalent trabecular bone mass and cortical bone thickness of non-fractured femurs (Supplemental Fig. 4d, e ). Unlike Ecsit Prx1 mice, tamoxifen-treated Ecsit Prx1-ERT/GFP mice displayed normal periosteal and callus formation and fracture unionization in the fractured sites (Supplemental Fig. 4b, f, g ). These results demonstrate that inducible deletion of Ecsit in Prx1 + skeletal progenitors in adult mice does not affect bone fracture healing and homeostasis. Thus, impaired fracture healing seen in Ecsit Prx1 mice may result from pre-existing skeletal phenotypes and/or alteration of skeletal progenitor population during early skeletal development. However, it cannot be fully excluded that inadequately complete deletion of Ecsit in this system contributes to the lack of a phenotype observed. Taken together, ECSIT-mediated mitochondrial functions play critical roles in osteogenic commitment and differentiation of skeletal progenitors during early skeletal development. ECSIT controls mitochondrial OXPHOS in skeletal progenitors Despite the original identification of ECSIT as a key regulator of NF-κB signaling downstream of pro-inflammatory receptors, Toll-like receptor (TLR) and interleukin (IL)-1β [38] , [39] , transcriptome analysis showed an enrichment of genes associated with metabolic pathways and mitochondrial function, not the NF-κB pathway in cKO Prx1 + skeletal cells (Fig. 2a, b ). Specifically, expression of the genes involved in mitochondrial CI biogenesis and OXPHOS was markedly downregulated in the absence of Ecsit while there was little to no altered expression in glucose and glutamine metabolism (Fig. 2b ). This is consistent with previous reports demonstrating ECSIT as a key component of the MCIA complex that controls the stability of CI subunits [31] , [32] , [33] . To directly test the role of ECSIT in mitochondrial OXPHOS, the expression of mitochondrial CI, II, III, IV, and V subunit proteins in the OXPHOS pathway was examined in WT and cKO Prx1 + skeletal progenitors, demonstrating that expression of core CI subunit proteins, including ND6, NDUFB8 and NDUFS3, was ablated in the absence of Ecsit while Ecsit deletion minimally affected the expression of proteins in other mitochondrial complexes (Fig. 2c , left). Similarly, Ecsit -deficiency significantly reduced expression of NDUFAF1, a key component of the MCIA complex [32] , [33] (Fig. 2c , right), suggesting the importance of ECSIT in stabilizing the components of CI and MICA complexes in Prx1 + skeletal progenitors. Accompanying our transcriptome analysis that show little to no enrichment of genes associated with mitochondrial biogenesis (Fig. 2b ), mRNA and protein levels of Atf5 [40] , [41] and Hsp90 [42] , [43] were largely intact in the absence of Ecsit (Fig. 2c , Supplemental Fig. 5a ). Of note, expression of Lc3b and Pink1 [44] , key regulators of mitophagy, was markedly increased in cKO Prx1 + skeletal progenitors (Fig. 2c ), suggesting enhanced mitophagy activity. These results suggest that Ecsit deletion in Prx1 + skeletal progenitors destabilizes the components of the MCIA and CI complexes while enhancing mitophagy activity. Accordingly, cKO Prx1 + skeletal progenitors displayed a significant decrease in mitochondrial numbers and transmembrane potential (Fig. 2d ), in the ratio of mitochondrial to nuclear DNA levels (Fig. 2e ), and in ATP production (Fig. 2f ). Along with a decrease in basal and maximal mitochondrial oxygen consumption (Fig. 2g ), cKO Prx1 + skeletal progenitors failed to respond to mitochondrial respiratory modulators, demonstrating the nearly complete absence of oxygen consumption rates (OCR, Fig. 2h ). Of note, the glycolytic proton efflux rate was markedly upregulated in these cells, as shown by greater extracellular acidification rate (ECAR, Fig. 2i ). However, enhanced glycolysis was incapable of compensating for the reduced ATP production by the damaged mitochondrial OXPHOS. In contrast to the involvement of glucose metabolism in RUNX2-mediated osteogenesis [45] , expression and transcription activity of RUNX2 were largely intact in cKO Prx1 + skeletal progenitors (Supplemental Fig. 5b, c ), suggesting that ECSIT-mediated mitochondrial oxidative metabolism is dispensable for RUNX2-mediated osteogenesis. Fig. 2: Ecsit -deficiency in skeletal progenitors impairs mitochondrial OXPHOS. a , b Gene ontology analysis showing biological processes with gene enrichment in cKO vs WT skeletal progenitors ( a ). Gene set enrichment analysis (GSEA) showing the enrichment of genes involved in OXPHOS, CI biogenesis, glycolysis, glutamine metabolism, and IKK-NFκB signaling ( b ). c Immunoblot analysis showing protein levels in cKO and WT skeletal progenitors. GAPDH was used for a loading control. d MitoTracker and TMRE staining (red) of GFP-expressing cKO and WT skeletal progenitors (green). DAPI was used for nuclear staining ( left ). The signal intensity of the stained cells was quantified using ImageJ software ( right ). (MitoTracker (WT), n = 6; MitoTracker (cKO), TMRE (WT, cKO), n = 5). e RT-PCR analysis showing the ratio of mitochondrial DNA (mtDNA, Ndufv1) to nuclear DNA (nDNA, 18s) in cKO and WT skeletal progenitors ( n = 4). f Intracellular ATP levels in cKO and WT skeletal progenitors were measured by colorimetric analysis ( n = 9). g – i . Seahorse assay showing a real time oxygen consumption rate (OCR, g–h ) and extracellular acidification rate (ECAR, i ) of cKO and WT skeletal progenitors before and after the addition of mitochondrial inhibitors ( n = 46). j Diagram of constructs for ECSIT-full length and the mutant lacking mitochondrial localization sequence (MLS, 1-47 aa). A FLAG epitope tag was inserted into the C-terminus of ECSIT cDNA ( top ). Immunoblot analysis showing mitochondrial fractionation of FLAG-ECSIT proteins in cKO skeletal progenitors. (bottom) . T total, S soluble, M mitochondrial fraction. k Immunoblot analysis showing expression of FLAG-ECSIT proteins in AAV-transduced cKO skeletal progenitors. l, m MitoTracker or TMRE staining of vector control or FLAG-ECSIT-expressing cKO and WT skeletal progenitors and quantification of deep red signal intensity ( l ). AAV-transduced cells were cultured under osteogenic conditions and ALP activity and osteogenic gene expression were assessed ( m , n = 4). A two-tailed unpaired Student’s t -test for comparing two groups ( d , e , f , g ) or ordinary one-way ANOVA with Dunnett’s multiple comparisons test ( l , m ). ( d – i , l – m ; data represent mean ± SD). Data ( e , f , g , m ) are representative of three independent experiments. Scale bars = d (left), l , 10 μm. Full size image Since ECSIT is localized on the membrane of mitochondria via an N-terminal mitochondria localization sequence (MLS, 1–48 aa) [32] , [46] , to investigate mechanistic actions of ECSIT in regulating mitochondrial OXPHOS, cKO Prx1 + skeletal progenitors were reconstituted with FLAG-tagged ECSIT full length (ECSIT-FL) or a MLS-deletion mutant (ECSIT-ΔMLS) that failed to localize to mitochondria via rAAV-mediated delivery (Fig. 2j ). Enforced expression of ECSIT-FL, not the ECSIT-ΔMLS mutant, reversed alterations in expression of the CI subunit NDUFS3, mitochondrial numbers and transmembrane activity, and osteogenic potential in cKO Prx1 + skeletal progenitors (Fig. 2k–m ). Thus, mitochondrial ECSIT regulates CI assembly and mitochondrial OXPHOS in Prx1 + skeletal progenitors, which in turn determines the osteogenic commitment and differentiation of skeletal progenitors. To confirm these findings in vivo, a bone-targeting rAAV was used to express FLAG-tagged ECSIT-FL and ECSIT-ΔMLS proteins in Ecsit Prx1 mice (Fig. 3a ). Given our previous report showing high transduction efficiency of the AAV9 serotype in osteoblast-lineage cells in vivo [47] , systemic delivery of AAV9 vector expressing mCherry to P1 Prx1;Rosa mT/mG neonates was effective in transducing GFP-expressing Prx1 + osteoblast-lineage cells, including skeletal progenitors, osteoprogenitors, and mature osteoblasts, in both trabecular and cortical compartments of long bones in addition to lung, heart, liver, kidney, and skeletal muscle (Fig. 3b, c ). AAV-mediated expression of FLAG-tagged ECSIT-FL and ECSIT-ΔMLS proteins in the femur and liver was confirmed (Fig. 3f , Supplemental Fig. 6 ). Remarkably, enforced expression of ECSIT-FL, but not a vector control or ECSIT-ΔMLS, markedly improved the survival rates of Ecsit Prx1 mice (Fig. 3d ). The osteogenic activity of Ecsit Prx1 skeletal progenitors was recovered by ECSIT-FL expression (Fig. 3f–h ), leading to recovery of bone formation and regeneration activity at multiple anatomic compartments. This led to an almost complete rescue of skeletal deformities in Ecsit Prx1 forelimbs and hindlimbs (Fig. 3e ) and abnormal bone marrow compartment (Fig. 3f , left) and impaired fracture healing and periosteal bone formation of Ecsit Prx1 long bones (Fig. 3g, h ). However, none of these phenotypes were improved by AAV-mediated expression of ECSIT-ΔMLS (Fig. 3d–h ). As expression of ECSIT-FL, not ECSIT-ΔMLS, restored OCN + mature osteoblasts and osteoblast-supporting CD31 + EDMC + type H endothelium [48] in the fracture callus of Ecsit Prx1 long bones, fracture healing progressed normally in these mice (Fig. 3g, h ). Restoring ECSIT levels in Prx1 + osteoblast-lineage cells, including skeletal progenitors, osteoprogenitors, and mature osteoblasts, reverses skeletal defects and retrieves bone regeneration during fracture in Ecsit Prx1 mice. Thus, ECSIT-mediated regulation of mitochondrial OXPHOS in skeletal progenitors is crucial for bone accrual, fracture repair, and bone marrow niche maintenance during early skeletal development. Fig. 3: AAV-mediated expression of ECSIT reverses Ecsit Prx1 skeletal phenotypes. a Diagram summarizing the study and treatment methods. A single dose of 2 x 10 11 genome copies (GCs) of rAAV9 vectors carrying control vector or FLAG-ECSIT constructs was injected into P1 Ecsit Prx1 neonates via the facial vein and musculoskeletal phenotypes were assessed 21 days post-injection (created with biorender.com). b Single dose of 2 x 10 11 GCs of rAAV9 carrying mCherry was injected into P0 Prx1;Rosa26 mTmG neonates via facial vein and mCherry expression was monitored by IVIS-100 optical imaging 21 days post-injection. c rAAV9 vector carrying mCherry was injected into Prx1;Rosa26 mTmG neonates and 21 days later, mCherry expression was assessed by fluorescence microscopy of cryo-sectioned femurs. d Survival rate of AAV-treated Ecsit Prx1 mice up to 21 days post-injection ( n = 6). e MicroCT analysis of the forelimbs (left) and hindlimbs (right) of P21 AAV-treated Ecsit fl/fl and Ecsit Prx1 mice ( n = 5–8). f Longitudinal sections of P21 AAV-treated Ecsit fl/fl and Ecsit Prx1 femurs were stained for H&E ( left ) or immunostained for OCN ( middle ) or FLAG-ECSIT ( right ). Blue lines indicate the bone marrow area. g H&E staining ( left ) or immunofluorescence for CD31, EDMC, or OCN ( middle, right ) of diaphyseal cortical bones of P21 AAV-treated Ecsit fl/fl and Ecsit Prx1 femurs. Blue lines indicate periosteum. h H&E staining ( top ) or immunofluorescence for CD31, EDMC (VEC, n = 7; ECSIT-FL, n = 8, ECSIT-MLS, n = 6), or OCN ( n = 6, middle, bottom ) of fracture sites of P21 AAV-treated Ecsit fl/fl and Ecsit Prx1 femurs. Immunofluorescence intensity was quantified using ImageJ software. An ordinary one-way ANOVA with Dunnett’s multiple comparisons test ( h ; error bars, data represent mean ± SD). Data are representative of three independent experiments. Scale bars = c , 50 μm; e , 1 mm; f , h , 100 μm; g , 75 μm. Full size image ECSIT is dispensable of mitochondrial OXPHOS in committed skeletal cells Since ECSIT is highly expressed in osterix (OSX) + committed osteoprogenitors and dentin matrix acidic phosphoprotein 1 (DMP1) + mature osteoblasts and osteocytes (Figs. 1 a and 4a ), the role of ECSIT in these cells were examined using conditional deletion with OSX-cre ( Ecsit Osx ) or DMP1-cre ( Ecsit Dmp1 ) mice. mRNA and protein levels of Ecsit in these mice were examined by RT-PCR, immunoblot, and immunohistochemistry analyses, demonstrating lack of Ecsit expression (Fig. 4b, d, g ). Remarkably, unlike Ecsit Prx1 mice, little to no gross skeletal phenotypes were seen in two-month-old Ecsit Osx and Ecsit Dmp1 mice. Bone morphology, trabecular bone mass, and cortical bone thickness were all normal in the long bones of these mice (Fig. 4c, e , Supplemental Fig. 7 ). In addition, osteogenic differentiation and bone fracture healing were largely intact in the absence of Ecsit (Fig. 4f , Supplemental Fig. 8 ). These results suggest that ECSIT function is dispensable for the development of committed osteoblast-lineage cells, including Osx + osteoprogenitors and Dmp1 + mature osteoblasts and osteocytes. Fig. 4: Ecsit Osx and Ecsit Dmp1 mice show no skeletal phenotype and intact mitochondrial function. a GFP-expressing Osterix (OSX)-, DMP1-lineage cells residing in the diaphyseal periosteum of P1 Osx-EGFP and DMP1-cre;Rosa26 mTmG mice, respectively, were monitored by fluorescence microscopy. m: muscle, bm: bone marrow. b , d mRNA levels of Ecsit in tibia was examined by RT-PCR ( n = 4, left ). Immunohistochemistry showing ECSIT expression in 2-month-old Ecsit Osx , Ecsit Dmp1 , and littermate control femurs ( right ). p: periosteum, tb: trabecular bone, c: cortical bone. Red arrows indicate Osx + or Dmp1 + lineage osteoblasts or osteoctyes. c , e MicroCT analysis showing 3D-reconstruction images of hindlimbs, femoral trabecular and cortical bones of 2-month-old Ecsit Osx , Ecsit Dmp1 and littermate control mice ( left ), and the relative quantification of trabecular bone mass (Osx-cre, Ecsit Osx , n = 8; Ecsit fl/fl , n = 7; Ecsit Dmp1 , n = 5) and cortical bone thickness (Osx-cre, n = 8; Ecsit Osx , n = 7; Ecsit fl/fl , n = 6; Ecsit Dmp1 , n = 4, right ). Osx-cre limbs were used as controls for Ecsit Osx mice. f MicroCT analysis showing sagittal and transverse views of fracture sites of 2-month-old Osx-cre , Ecsit Osx , and Ecsit fl/fl femurs 10 weeks after the surgery, and the relative quantification of fracture union rates ( n = 5). g – i Osteoprogenitors and osteoblasts were isolated from Osx-cre and Ecsit Osx calvaria and Ecsit fl/fl and Ecsit Dmp1 long bones, respectively. Immunoblot analysis showing protein levels in the isolated cells. GAPDH was used as a loading control ( g ). A ratio of mtDNA (Ndufv1) to nDNA (18s) was assessed by RT-PCR ( n = 4, h ). Fluorescence microscopy shows MitoTracker- and TMRE-stained cells ( i, left ) and relative quantification of MitoTracker- ( n = 5, i , middle ) and TMRE-red signal intensity ( n = 5, i , right ). A two-tailed unpaired Student’s t -test for comparing two groups ( b , c , d , e , h , i ; error bars, data represent mean ± SD) or a Fisher’s exact test ( f , p > 0.9999) was applied. Data are representative of three independent experiments. Scale bars = a , 75 μm; b , d , 100 μm; c , e ( left, top ) 2 mm; c , e ( left, middle and bottom ), 100 μm; f , 1 mm; i ( left ), 25 μm. Full size image To gain insights on this mechanism, mitochondrial OXPHOS was examined in Ecsit Osx osteoprogenitors and Ecsit Dmp1 mature osteoblasts. Unlike Ecsit prx1 skeletal progenitors, expression of the CI protein NDUFS3, ND6, and NDUFB8, and the MCIA subunit NDUFAF1 (Fig. 4g ), the ratio of mitochondrial DNA to nuclear DNA (Fig. 4h ), mitochondrial numbers and transmembrane potential (Fig. 4i ) were all intact in these cells, suggesting that ECSIT function is dispensable for mitochondrial OXPHOS in Osx + committed osteoprogenitors and Dmp1 + mature osteoblasts and osteocytes. Notably, while a similar decrease in ECSIT expression was observed among Ecsit Prx1 skeletal progenitors, Ecsit Osx osteoprogenitors, and Ecsit Dmp1 osteoblasts, only Ecsit Prx1 cells showed a significant decrease in NDUFS3 expression (Supplemental Fig. 9 ). However, it cannot be fully excluded that inadequately deletion of Ecsit in osteoblasts may contribute to the lack of an observed phenotype. Thus, the role of ECSIT in controlling mitochondrial oxidative metabolism is context- and tissue-dependent. Ecsit deficiency in skeletal progenitors induces muscle atrophy Accompanying the onset spontaneous fractures in Ecsit Prx1 mice is an onset of myopathy and muscle atrophy. Specifically, the size and weight of skeletal muscles, including tibialis anterior (TA) and gastrocnemius (GA) muscles, were dramatically decreased (Fig. 5a, b , Supplemental Fig. 10a ). While muscle structure of Ecsit Prx1 neonates is grossly normal after birth (Fig. 5c , Supplemental Fig. 10b ), Ecsit Prx1 mice gradually developed severe degeneration of skeletal muscle, as evident by significant decrease in mature myofibers, extracellular matrix in the interstitial space, and the expression of mature myoblast genes (Fig. 5d, e , Supplemental Fig. 10c ). Despite a substantial decrease in total myocyte numbers in Ecsit Prx1 mice, the frequency of skeletal muscle-resident satellite cells [49] (β-integrin + CXCR4 + Sca1 - CD45 - CD11b - TER119 - ) and mesenchymal progenitors [50] (Sca1 + integrin α7 - CD45 - CD31 - ) was dramatically increased in Ecsit Prx1 muscle (Fig. 5f , Supplemental Fig. 11 ), indicating a defect in myoblast differentiation, but not the maintenance of muscle-resident stem cells. Of note, this phenotype does not result from the intrinsic effects of Ecsit deficiency in muscle cells, as shown by intact expression of Ecsit mRNA and protein in Ecsit Prx1 muscle (Fig. 5d, e ). This is accompanied by fluorescence microscopy showing little to no Prx1-cre driven reporter activity in skeletal muscle cells of Prx1-cre;Rosa26 mT/mG mice (Fig. 5g ). To directly test this, mice with targeted deletion of Ecsit in myoblast precursors ( Ecsit Myf5 ) were generated, demonstrating little to no gross phenotypes in the skeletal muscle, bone, and bone marrow (Fig. 5h ). Likewise, the expression of mature myoblast genes in the skeletal muscle of these mice was also normal (Fig. 5i ). Additionally, primary human myoblast progenitors (17Ubic) [51] with Ecsit knockdown were cultured under myogenic conditions, demonstrating no effect of Ecsit -deficiency on myoblast differentiation (Fig. 5j ). As seen in Osx + committed osteoprogenitors and Dmp1 + mature osteoblasts (Fig. 4g ), deletion of Ecsit in myoblast progenitors did not affect expression of CI protein NDUFS3, the ratio of mitochondrial DNA to nuclear DNA, mitochondrial numbers and transmembrane potential while these cells showed a mild reduction in the MCIA subunit Ndufaf1 (Fig. 5k, l ). These results suggest that ECSIT function is dispensable for mitochondrial OXPHOS for ATP production during myoblast differentiation. Thus, Ecsit deletion in Prx1 + skeletal progenitors, not muscle cells, is responsible for muscle atrophy in Ecsit Prx1 mice. Fig. 5: Ecsit Prx1 mice display skeletal muscle atrophy. a Graph shows the kinetics of fracture incidence and skeletal muscle weight of Ecsit Prx1 and Ecsit fl/fl mice ( n = 5, left ). Representative macroscopic images of the gastrocnemius (GA) muscle at the age of P0 and P10 ( right ). b Quantification of skeletal muscle weight ( left ) and a ratio of skeletal muscle weight to body weight ( right ) are displayed ( n = 5). c , d P0 ( c ) or P15 ( d ) Ecsit Prx1 and Ecsit fl/fl tibialis anterior (TA) muscles were stained for H&E or immunostained for MF20, COL1α1, or ECSIT. e mRNA levels of myogenic genes in P10 Ecsit Prx1 and Ecsit fl/fl TA muscles ( n = 16). f Total cell number ( n = 5) and flow cytometry analysis showing the frequency of muscle satellite cells (MuSCs) and skeletal muscle resident stem/progenitor cells ( Ecsit fl/fl , n = 9, Ecsit Prx1 , n = 5) in P10 Ecsit Prx1 and Ecsit fl/fl GA muscles. Supplemental Fig. 11 demonstrates the gating strategy for this analysis. g GFP-expressing Prx1 + skeletal cells in P3 Prx1-cre;Rosa26 mTmG GA muscle. Red: Prx1 - bone marrow and muscle. h , i Tibialis anterior muscles or femurs of E21 Ecsit Myf5 and Ecsit fl/fl embryos were stained for H&E, Von Kossa, or immunostained for MF20 ( h ). mRNA levels of Ecsit and myoblast genes in the skeletal muscle ( i , Ecsit fl/fl , n = 4−5; Ecsit Myf5 , n = 3). j Human 17Ubic myoblasts expressing control (shCtrl) or ECSIT shRNA (shECSIT) were cultured under myogenic conditions. 6 days later, expression of MF20 (green) and myogenic genes was assessed ( n = 4). k , l Protein levels of NDUFAF1, ECSIT and NDUFS3 ( k , left ) or the ratio of mtDNA (Ndufv1) to nDNA (18s, k , right ) in shCtrl or shECSIT-expressing 17Ubic cells. Fluorescence microscopy shows MitoTracker- and TMRE-stained cells and relative quantification of deep red signal intensity ( n = 6, l ). A two-tailed unpaired Student’s t -test for comparing two groups ( b , e , f , i , j , k , l ; error bars, data represent mean ± SD). Data are representative of three independent experiments. Scale bars = c , d , 60 μm; g , 75 μm; h , 30 μm; j , 100 μm; l , 10 μm. Full size image To determine how skeletal fracture could lead to muscle atrophy, the migration of GFP-expressing Ecsit Prx1 skeletal progenitors into skeletal muscle was monitored at fracture sites. Wild-type mice undergoing fracture did not experience muscle degeneration, showing normal callus formation at 7- and 14-days post-fracture, and restriction of wild-type Prx1- lineage skeletal cells to the callus and not adjacent skeletal muscle (Fig. 6a ). On the other hand, Ecsit Prx1 mice showed abnormal callus development and fibrotic tissue at fracture sites and failed to form periosteum, where Ecsit Prx1 skeletal progenitors migrated into the skeletal muscle and induced degeneration of myofibers (Fig. 6b ). In non-fractured long bone showing normal muscle structure, Ecsit Prx1 skeletal progenitors were only detected inside the bone (Fig. 6c ). Thus, impaired fracture healing and periosteal formation allow migration of Ecsit Prx1 skeletal progenitors to adjacent skeletal muscle, resulting in muscle atrophy. To directly test this hypothesis, conditioned media (CM) harvested from WT or cKO Prx1 + skeletal progenitors were added to cultures of human myoblast progenitors (17Ubic). These studies demonstrated a significant reduction in myoblast differentiation in the presence of cKO-CM compared to WT-CM (Fig. 6d ). Transcriptome and RT-PCR analyses of FACS-sorted WT and cKO Prx1 + skeletal progenitors and SSCs revealed elevated levels of the soluble myogenic suppressor TGF-β1 [52] , [53] in cKO cells (Fig. 6e, f ). Since TGF-β1 expression was unchanged in satellite cells (MuSCs) isolated from the skeletal muscle of Ecsit Prx1 mice and Ecsit -deficient myoblast progenitors (Fig. 6f, g ), cKO Prx1 + skeletal progenitors and SSCs, not MuSCs and myoblast progenitors, are likely to be major contributors of TGF-β1 expression in skeletal muscle. Accordingly, the TGF-β1 inhibitor SB-431542 almost completely reversed the ability of cKO-CM to suppress myoblast differentiation (Fig. 6d ). Since the TGF-β pathway plays a role in the pathogenesis of skeletal muscle myopathies and its inhibition is considered for the treatment of skeletal muscle fibrosis [54] , TGF-β1 is likely to be an important factor mediating the myoblast suppressive activity of Ecsit Prx1 skeletal progenitors, though other pathways may contribute as well. Fig. 6: Ecsit Prx1 skeletal progenitors induce skeletal muscle degeneration. a X-radiography ( left ) and H&E staining ( right ) of P14 Ecsit; Prx1 Rosa26 mTmG tibias with spontaneous fractures and 6-week-old Prx1;Rosa26 mTmG tibias 14 days post-fracture surgery. b Fluorescence microscopy showing GFP-expressing Prx1 + skeletal cells in P7 or P14 Ecsit; Prx1 Rosa26 mTmG tibias with spontaneous fracture and 6-week-old Prx1;Rosa26 mTmG tibias 7- or 14-days post-fracture surgery. Red: Prx1 - tissues. c Non-fractured sites in P0 ( left ) or P15 ( right ) Ecsit; Prx1 Rosa26 mTmG femurs, demonstrating intact skeletal muscle structure. Green: Prx1 + skeletal cells. Red: Prx1 - bone marrow and muscle. d Human 17Ubic myoblasts were cultured under myogenic conditions in the presence of conditioned medium (CM) harvested from the culture of FACS-sorted Ecsit; Prx1 Rosa26 mTmG (cKO) and Prx1;Rosa26 mTmG (WT) skeletal progenitors. 5 days later, expression of MF20 (green) and myogenic genes was assessed ( n = 4). Alternatively, cells were treated with the TGF-β1 inhibitor SB431542. e RNA sequencing was performed on FACS-sorted Ecsit; Prx1 Rosa26 mTmG (cKO) and Prx1;Rosa26 mTmG (WT) skeletal progenitors. A volcano plot shows the gene expression for up/downregulated genes in cKO cells relative to WT cells. f mRNA levels of Tgf-β1 in FACS-sorted skeletal progenitors ( left ), SSCs ( middle ), or skeletal muscle satellite cells (MuSCs, right ) ( n = 4). g mRNA levels of Tgfβ1 in 17Ubic myoblast progenitors expressing control (shCtrl) or ECSIT shRNA (shECSIT) ( n = 4). h , i AAV-treated Ecsit fl/fl and Ecsit Prx1 TA muscles (P21) were stained for H&E ( h, top ) or immunostained for MF20 ( h, bottom ). H&E staining demonstrate intact cortical bone, periosteum, and skeletal muscle in Ecsit Prx1 mice expressing FLAG-tagged ECSIT-FL, not ECSIT-ΔMLS ( i ). White lines indicate the barrier between bone and skeletal muscle. j mRNA levels of Tgf-β1 in vector control or FLAG-ECSIT-expressing cKO and WT skeletal progenitors ( n = 4). A two-tailed unpaired Student’s t-test for comparing two groups ( f, g ) or ordinary one-way ANOVA with Dunnett’s multiple comparisons test ( d, j ) ( d, f, i , data represent mean ± SD). Data are representative of three independent experiments. Scale bars = a , c , 200 μm; b , d , 100 μm; h , 75 μm; i , 20 μm. Full size image Intravenous administration of P1 Ecsit Prx1 neonates with bone-targeting rAAV9 expressing FLAG-tagged ECSIT-FL, not ECSIT-ΔMLS mutant, almost completely recovered degeneration of skeletal muscle (Fig. 6h ). This was accompanied with little to no migration of Ecsit Prx1 skeletal progenitors expressing ECSIT-FL, not ECSIT-ΔMLS mutant, to the skeletal muscle (Fig. 6i ). Finally, enforced expression of ECSIT-FL markedly decreased TGF-β transcription in FACS-sorted cKO Prx1 + skeletal progenitors while TGF-β expression was partially reversed by ECSIT-ΔMLS mutant (Fig. 6j ), suggesting the presence of additional functional domain(s) within Ecsit regulating TGF-β expression. Thus, impaired OXPHOS in skeletal progenitors is likely to be responsible for muscle atrophy seen in Ecsit Prx1 mice. Taken together, ECSIT-mediated regulation of mitochondrial oxidative metabolism is a key determinant of the osteogenic commitment and differentiation of Prx1 + skeletal progenitors, governing musculoskeletal development and bone marrow niche functions. Our study provides in vivo evidence showing the importance of mitochondrial oxidative metabolism in determining osteogenic commitment and differentiation of skeletal progenitors during early skeletal development. Despite emerging evidence suggesting an association of mitochondrial dysfunction and high oxidative stress in skeletal cells with skeletal disorders [17] , only few genetic models with mitochondrial OXPHOS defects have been successfully generated due to either embryonic lethality or the absence of any relevant phenotypes. Herein, we generated a mouse model with CI deficiency by conditionally deleting the key CI assembly factor Ecsit in various musculoskeletal cells. Deletion of Ecsit in Prx1 + skeletal progenitors disrupts mitochondrial OXPHOS for ATP production while enhancing glucose metabolism as a compensatory mechanism. Lack of OXPHOS activity ablates the osteogenic potential of skeletal progenitors, resulting in defects in skeletal development, bone marrow niche maintenance, and bone fracture repair. Surprisingly, breakdown of this regulatory circuit leads to the infiltration of Prx1 + skeletal progenitors into adjacent muscle, which induces myopathy mediated by TGF-β1 (Supplemental Fig. 12 ). This unexpected finding indicates that OXPHOS defects or TGF-β1 may be implicated in paired skeletal fragility/myopathy disorders, and there may be potential therapeutic targets in this context. Intriguingly, despite the requirement of mitochondrial localization of Ecsit in regulating mitochondrial oxidative metabolism in Prx1 + skeletal progenitors, our findings that cytosolic Ecsit (Ecsit-ΔMLS) can partially improve survival of Ecsit Prx1 mice and TGF-β1 expression in Ecsit Prx1 skeletal progenitors suggest the presence of additional functional domain(s) within Ecsit regulating survival and TGF-β1 expression. Further studies will be necessary to identify these functional domains in Prx1 + skeletal progenitors. Glucose and glutamine metabolism and mitochondrial OXPHOS have been known as major pathways of energy metabolism regulating the production of ATP in osteoblast-lineage cells [24] . In particular, glucose and glutamine metabolism are prominent metabolic features of committed osteoblast-lineage cells [55] , [56] , [57] , [58] and integral to collagen production and mineralizing activity by generating ATP and intermediate metabolites [59] , [60] . In contrast to our findings that ECSIT-mediated mitochondrial OXPHOS provides an energy source crucial to the osteogenic commitment and differentiation of Prx1 + skeletal progenitors during skeletal development, glutamine metabolism mainly contributed to biosynthesis and redox homeostasis, but not energy production, during bone remodeling. Of note, since amino-acid-transaminase-derived αKG is the critical downstream glutamine metabolite regulating proliferation of skeletal progenitors [29] , cell proliferation rates were largely not altered in Ecsi Prx1 skeletal progenitors with normal glutamine metabolism. Intriguingly, despite extensive studies showing that glucose is a major nutrient for osteoblast development, mice lacking the glucose transporter Glut1 in Prx1 + skeletal progenitors displayed impaired cartilage development without any alteration in skeletal mineralization [28] . This suggests that glycolysis is critical for chondrogenesis, not osteogenesis, of Prx1 + skeletal progenitors during skeletal development. Notably, Ecsit -deficiency in Prx1 + skeletal progenitors enhanced glucose metabolism as a compensatory mechanism while cartilage development occurred normally in Ecsi Prx1 mice. Thus, our data implies that mitochondrial OXPHOS, not glucose or glutamine metabolism, is the major energy-driving force for osteogenesis in skeletal progenitors and that it is, therefore, critical for skeletal development and the maintenance of musculoskeletal integrity. We note that reduced mitochondrial mass in Ecsi Prx1 skeletal progenitors also potentially results in a broader set of cellular abnormalities than just decreased ATP synthesis, as many TCA cycle metabolites, such as acetyl-CoA and α-ketoglutaric acid, have direct roles in lipid synthesis, protein acetylation, histone demethylation, and other processes [29] , [61] , [62] . Since ECSIT function is dispensable for Osx + committed osteoprogenitors and Dmp1 + mature osteoblasts and terminally differentiated osteocytes, glycolysis may offset this as glycolysis is the primary metabolic pathway for ATP production during the differentiation of committed osteoblast-lineage cells [59] . Further studies will be necessary to determine how ECSIT controls mitochondrial oxidative metabolism and osteogenic development in a context and tissue-dependent manner. Additional further studies are warranted to define the precise mechanisms by which mitochondrial OXPHOS impacts skeletal progenitors through other mitochondrial regulatory mechanisms, such as mitochondrial biogenesis, the degradation of damaged mitochondria via mitophagy, reactive oxygen species (ROS) generation, and mtDNA replication and/or transcription. The unexpected finding that mitochondrial defects lead Ecsit Prx1 skeletal progenitors to infiltrate into muscle and mediate pathogenic TGF-β1 secretion, provides a new potential explanation for a number of clinical disorders that pair prominent or primary skeletal phenotypes with myopathy. For instance, Kearns Sayre Syndrome displays linked skeletal and myopathy phenotypes due to mitochondrial dysfunction, raising the possibility that the myopathy may be in part secondary to pathogenic infiltration of skeletal progenitors into adjacent muscle [20] . rAAVs have been considered the most promising viral vector for gene therapy [63] , as they have a clinical track record of being well tolerated and have the potential to efficiently mediate genetic modifications that can persist for years after a single treatment. Remarkably, AAV-mediated expression of full length Ecsit almost completely restored impaired mitochondrial OXPHOS and osteogenic potentials of Ecsit Prx1 progenitors, preventing musculoskeletal deformities of Ecsit Prx1 mice. Thus, our findings provide proof-of-concept demonstration for gene therapy of developmental skeletal disorders. Collectively, this study reveals a previously unappreciated role of mitochondrial oxidative metabolism in determining osteogenesis of skeletal progenitors and demonstrates a new gene therapy approach for mitochondrial diseases in the musculoskeletal system. Mice Mice were housed in a constant environment under a standard mouse chow diet (up to 5 mice per cage); ambient temperature of 21 ± 2 °C, circulating air, and constant humidity of 50 ± 10%, in a 12 h light, 12 h dark cycle. Mice were monitored every three days for the amount of their food and water intake and signs for distress. For signs of severe distress, including general malaise, severe cachexia, or more than 20% loss of body weight, humane euthanasia was performed in consultation with veterinary staff. Mice were euthanized in a carbon dioxide chamber, followed by cervical dislocation. Neonates were euthanized by decapitation. Ecsit fl/fl mice were generated as previously described and maintained on a C57BL/6J background [46] . Cre deleter mice (C57BL/6J) that express Cre recombinase under the control of the prx1 promoter (Prx1-cre), the osterix promoter (Osx-cre), and the dmp1 promoter (Dmp1-cre) were purchased from The Jackson Laboratory. To label Cre-expressing cells, Ecsit ; fl/fl Prx1-cre mice were further crossed with Rosa mT/mG cre reporter mice (C57BL/6J) [64] . Mouse genotypes were determined by PCR on tail genomic DNA and primer sequences are available upon request. Control littermates were used and analyzed in all experiments. A phenotypic summary of Ecsit Prx1 mice is described in Supplemental Table 1 . All animals were used in accordance with the NIH Guide for the Care and Use of Laboratory Animals and were handled according to protocols approved by the University of Massachusetts Medical School Institutional Animal Care and Use Committee (IACUC). Generation of rAAV vectors DNA sequences for ECSIT-FL and ECSIT-ΔMSL were synthesized as gBlocks, cloned into the intronic region of the pAAVsc-CB6-Egfp plasmid at the restriction enzyme sites (PstI and BglII) [65] , and packaged into an AAV9 capsid. rAAV production was performed by transient transfection of HEK293 cells, purified by CsCl sedimentation, titered by droplet digital PCR (ddPCR) on a QX200 ddPCR system (Bio-Rad) using the Egfp prime/probe set as previously described [47] , [65] . 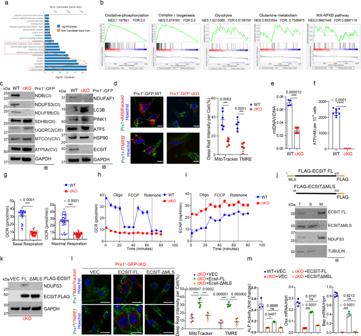Fig. 2:Ecsit-deficiency in skeletal progenitors impairs mitochondrial OXPHOS. a,bGene ontology analysis showing biological processes with gene enrichment in cKO vs WT skeletal progenitors (a). Gene set enrichment analysis (GSEA) showing the enrichment of genes involved in OXPHOS, CI biogenesis, glycolysis, glutamine metabolism, and IKK-NFκB signaling (b).cImmunoblot analysis showing protein levels in cKO and WT skeletal progenitors. GAPDH was used for a loading control.dMitoTracker and TMRE staining (red) of GFP-expressing cKO and WT skeletal progenitors (green). DAPI was used for nuclear staining (left). The signal intensity of the stained cells was quantified using ImageJ software (right). (MitoTracker (WT),n= 6; MitoTracker (cKO), TMRE (WT, cKO),n= 5).eRT-PCR analysis showing the ratio of mitochondrial DNA (mtDNA, Ndufv1) to nuclear DNA (nDNA, 18s) in cKO and WT skeletal progenitors (n= 4).fIntracellular ATP levels in cKO and WT skeletal progenitors were measured by colorimetric analysis (n= 9).g–i. Seahorse assay showing a real time oxygen consumption rate (OCR,g–h) and extracellular acidification rate (ECAR,i) of cKO and WT skeletal progenitors before and after the addition of mitochondrial inhibitors (n= 46).jDiagram of constructs for ECSIT-full length and the mutant lacking mitochondrial localization sequence (MLS, 1-47 aa). A FLAG epitope tag was inserted into the C-terminus of ECSIT cDNA (top). Immunoblot analysis showing mitochondrial fractionation of FLAG-ECSIT proteins in cKO skeletal progenitors.(bottom). T total, S soluble, M mitochondrial fraction.kImmunoblot analysis showing expression of FLAG-ECSIT proteins in AAV-transduced cKO skeletal progenitors.l, mMitoTracker or TMRE staining of vector control or FLAG-ECSIT-expressing cKO and WT skeletal progenitors and quantification of deep red signal intensity (l). AAV-transduced cells were cultured under osteogenic conditions and ALP activity and osteogenic gene expression were assessed (m,n= 4). A two-tailed unpaired Student’st-test for comparing two groups (d,e,f,g) or ordinary one-way ANOVA with Dunnett’s multiple comparisons test (l,m). (d–i,l–m; data represent mean ± SD). Data (e,f,g,m) are representative of three independent experiments. Scale bars =d (left), l, 10 μm. The sequences of gBlocks and oligonucleotides for ddPCR and are listed in Supplemental Table 2 . MicroCT, radiography, and skeletal preparation MicroCT was used for qualitative and quantitative assessment of trabecular and cortical bone microarchitecture and performed by an investigator blinded to the genotypes of the animals under analysis. Femurs excised from the indicated mice were scanned using a microCT 35 (Scanco Medical) with a spatial resolution of 7 μm. For trabecular bone analysis of the distal femur, an upper 2.1 mm region beginning 280 μm proximal to the growth plate was contoured. For cortical bone analysis of the femur and tibia, a midshaft region of 0.6 mm in length was used. MicroCT scans of forelimbs and hindlimbs were performed using isotropic voxel sizes of 12 μm. 3D reconstruction images were obtained from contoured 2D images by methods based on distance transformation of the binarized images. All images presented are representative of the respective genotypes ( n = 5–8). X-radiographic images of whole body and hindlimbs were taken by the Trident Specimen Radiography System (Hologic, Inc.). Skeletons were prepared for gross morphology analysis using the McLeod method, as previously described [66] . Briefly, mice were sacrificed, skinned, eviscerated, and fixed in 95% ethanol for one day. Then, skeletons were stained by alizarin red s and alcian blue solutions (Sigma, A3157) and sequentially cleared in 1% potassium hydroxide. All images presented are representative of the respective genotypes ( n = 3–5). Histology, immunofluorescence, and immunohistochemistry Histological analysis was performed on liver and hindlimbs, and skeletons and skeletal muscles were dissected from mice fixed in 4% PFA for one day, and decalcified by daily changes of 15% tetrasodium EDTA for one to two weeks. Tissues were dehydrated by passage through an ethanol series, cleared twice in xylene, embedded in paraffin, and sectioned at 5 μm thickness along the coronal plate from anterior to posterior. Decalcified femoral sections were stained with hematoxylin and eosin (H&E) or safranin O. Alternatively, intact hindlimbs containing bones and skeletal muscles were immediately fixed in ice-cold 4% paraformaldehyde solution for one day for histological analysis of skeletal muscles. Semi-decalcification was carried out for five days in 0.5 M EDTA pH 7.4 at 4 °C with constant shaking (age ≥1 week), and infiltration was followed with a mixture of 20% sucrose phosphate buffer for one day. All samples were embedded in a 50/50 mixture of 25% sucrose solution and OCT compound (Sakura) and cut into 10 μm thick cross sections using a cryostat (Leica Microsystems, USA). Immunofluorescence staining and analysis were performed, as described previously [8] . Briefly, after treatment with 0.2% Triton X-100 for 10 min, cryosections were blocked with 5% donkey serum at room temperature for 30 min and incubated overnight at 4 °C with primary antibody and then visualized with fluorescence-conjugated secondary antibody (1:400, Molecular Probes). Nuclei were counterstained with 4–6,diamidino-2-phenylindole (DAPI). An Olympus IX81 confocal microscope or Leica TCS SP5 II Zeiss LSM-880 confocal microscope or EVOS epifluorescence microscope was used to image samples. Osteocalcin (OCN, sc-365797, Santa Cruz Biotechnology, 1:100), ECSIT (HPA042979, Sigma,1:100), ECSIT (gifted from Dr. Sankar Gosh, Columbia University), NDUFS3 (43–9200, Invitrogen,1:100), CD31/PECAM-1 (AF3628, R&D systems, 1:50), Endomucin (sc-65495, Santa Cruz Biotechnology, 1:100), COL1A1 (A1352, ABclonal, 1:50), MF20 (AB_2147781, DSHB, 1:100) and anti-FLAG-tag (MA1-142-A488, Sigma-Aldrich, 1:100) were used for primary antibodies. For immunohistochemistry, paraffin sections were dewaxed and stained according to the manufacturer’s directions, using the Discovery XT automated IHC stainer (Ventana Medical Systems, Inc., Tucson, AZ, USA). CC1 standard (pH 8.4 buffer contained Tris/Borate/EDTA) and inhibitor D (3% H 2 O 2 , Endogenous peroxidase) were used for antigen retrieval and blocking, respectively. Sections were incubated with antibodies specific to ECSIT (A7804, ABclonal,1:200) for 40 min at 37 °C, and a secondary antibody for 20 min at 37 °C. 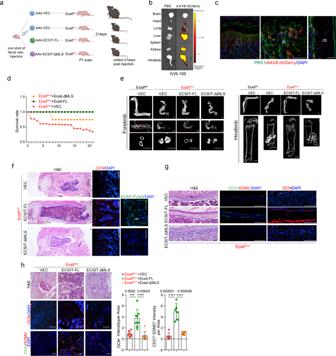Fig. 3: AAV-mediated expression of ECSIT reversesEcsitPrx1skeletal phenotypes. aDiagram summarizing the study and treatment methods. A single dose of 2 x 1011genome copies (GCs) of rAAV9 vectors carrying control vector or FLAG-ECSIT constructs was injected into P1EcsitPrx1neonates via the facial vein and musculoskeletal phenotypes were assessed 21 days post-injection (created with biorender.com).bSingle dose of 2 x 1011GCs of rAAV9 carrying mCherry was injected into P0Prx1;Rosa26mTmGneonates via facial vein and mCherry expression was monitored by IVIS-100 optical imaging 21 days post-injection.crAAV9 vector carrying mCherry was injected intoPrx1;Rosa26mTmGneonates and 21 days later, mCherry expression was assessed by fluorescence microscopy of cryo-sectioned femurs.dSurvival rate of AAV-treatedEcsitPrx1mice up to 21 days post-injection (n= 6).eMicroCT analysis of the forelimbs(left)and hindlimbs(right)of P21 AAV-treatedEcsitfl/flandEcsitPrx1mice (n= 5–8).fLongitudinal sections of P21 AAV-treatedEcsitfl/flandEcsitPrx1femurs were stained for H&E (left) or immunostained for OCN (middle) or FLAG-ECSIT (right). Blue lines indicate the bone marrow area.gH&E staining (left) or immunofluorescence for CD31, EDMC, or OCN (middle, right) of diaphyseal cortical bones of P21 AAV-treatedEcsitfl/flandEcsitPrx1femurs. Blue lines indicate periosteum.hH&E staining (top) or immunofluorescence for CD31, EDMC (VEC,n= 7; ECSIT-FL,n= 8, ECSIT-MLS,n= 6), or OCN (n= 6,middle, bottom) of fracture sites of P21 AAV-treatedEcsitfl/flandEcsitPrx1femurs. Immunofluorescence intensity was quantified using ImageJ software. An ordinary one-way ANOVA with Dunnett’s multiple comparisons test (h; error bars, data represent mean ± SD). Data are representative of three independent experiments. Scale bars =c, 50 μm;e, 1 mm;f,h, 100 μm;g, 75 μm. Subsequently, they were incubated in SA-HRP D for 16 min at 37 °C and then DAB + H 2 O 2 substrate for 8 min, followed by hematoxylin and bluing reagent counterstain at 37 °C. Reaction buffer (pH 7.6 Tris buffer) was used as washing solution. Stained samples were visualized using an Aperio virtual microscope (Leica Microsystems, USA) and images of the sample were analyzed by the Aperio image scope program (ver. 12.3.2.8013, Leica Microsystems, USA). Human myoblast and mouse osteoblast and osteoclast differentiation Human primary myoblasts 17Ubic were kindly gifted from Dr. Charles P Emerson at UMass Chan Medical school. Informed consent was obtained from the patients who donated tissue for the production of cell lines. IRB protocols were approved by UMass Chan Medical School (H00006581-10 and H00006581-11) and by Kennedy Krieger Institute (B0410080117). For human myoblast differentiation, human primary myoblasts 17Ubic [51] were cultured in growth medium (20% FBS,0.5% CEE and 1.2 mM CaCl 2 in Ham’s F10 medium) and plated into a collagen-coated 100 mm Petri-dish. To induce myogenic differentiation and fusion, cells were cultured in growth medium until >95% confluency and changed with differentiation medium (OPTI-MEM). Knockdown of ECSIT expression in 17Ubic cells was performed using lentivirus-mediated delivery of human ECSIT shRNA hairpins and knockdown efficiency was confirmed by immunoblotting. Alternatively, conditioned medium was harvested from cultured Ecsit ; +/+ Prx1-Cre;Rosa mT/mG or Ecsit ; fl/fl Prx1-Cre;Rosa mT/mG skeletal cells and added to 17Ubic cells. 6 days after myogenic culture (30% conditioned medium + 70% myogenic differentiation medium), myoblast differentiation was analyzed by immunofluorescence for MF20 and RT-PCR for myogenic gene expression. The ALK inhibitor SB-431542 (S4317) was purchased from Sigma-Aldrich and added to the culture at a final concentration of 1 µM. For mouse osteoblast differentiation, GFP-expressing Prx1 + skeletal cells were FACS-sorted from P1 Ecsit ; +/+ Prx1-Cre;Rosa mT/mG and Ecsit ; fl/fl Prx1-Cre;Rosa mT/mG neonates using cell surface markers (CD45 - Tie2 - Ter119 - ). 6 days after osteogenic culture, skeletal cells were fixed with10% neutral formalin buffer and stained with the solution containing Fast Blue (Sigma-Aldrich, FBS25) and Naphthol AS-MX (Sigma-Aldrich, 855) to assess alkaline phosphatase (ALP) activity. Subsequently, cells were washed and incubated with a solution containing 6.5 mM Na2CO3, 18.5 mM NaHCO 3 , 2 mM MgCl 2 , and phosphatase substrate (Sigma-Aldrich, S0942), and ALP activity was measured by spectrometer (BioRad). Finally, cell survival was analyzed by staining with Alamar Blue solution (DAL1100, Invitrogen). For osteoclast differentiation, bone marrow cells were flushed from long bones of two-month-old Ecsit fl/fl mice and cultured in the presence of 10 ng/ml M-CSF (R&D systems) to obtain bone marrow-derived macrophages (BMMs). Twenty-four hours later, the non-adherent cells were re-plated, cultured in the medium containing 20 ng/ml of M-CSF for 3 days, and then 10 ng/ml of RANKL were added to induce osteoclast differentiation. Twelve hours later, BMMs were treated with rAAV9 vectors expressing control vector or Cre recombinase, cultured in the presence of 20 ng/ml of M-CSF and 10 ng/ml of Rank ligand for 6 days, and osteoclast differentiation was analyzed by TRAP staining and RT-PCR analysis. Quantitative RT-PCR and immunoblotting Fresh tibialis anterior (TA) muscle and gastrocnemius (GA) muscle tissues were dissected and homogenized mechanically in QIAzol (QIAGEN) to isolate total RNA samples. cDNA was synthesized using the HighCapacity cDNA Reverse Transcription Kit from Applied Biosystems. Quantitative RT-PCR was performed using SYBR® Green PCR Master Mix (Applied Biosystems) with QuantStudio (TM) 6 Flex System (Applied Biosystems). The primers used for PCR are described in Supplemental Table 2 . For immunoblotting analysis, cells were lysed in TNT lysis buffer (50 mM Tris-HCl (pH 7.4), 150 mM NaCl, 1% Triton X-100, 1 mM EDTA, 1 mM EGTA, 50 Mm NaF, 1 mM Na 3 VO 4 , 1 mM PMSF, and protease inhibitor cocktail (Sigma-Aldrich), and protein amounts from cell lysates were measured using the DC protein assay (BioRad). Equivalent amounts of proteins were subjected to SDS-PAGE, transferred to Immunobilon-P membranes (Millipore), immunoblotted with antibodies specific to ECSIT (HPA042979, Sigma,1:1000), ECSIT (a gift from Dr. Sankar Gosh, Columbia University), NDUFS3 (43–9200, Invitrogen, 1:1000), PINK1 (BC100, Novus Biologicals, 1:1000), LC3B (2775S, Cell Signaling Technology, 1:1000), ND6 (NBP2–94464, Novus Biologicals, 1:1000), NDUFAF1 (PA5–59051, Thermofisher, 1:1000), HSP90 (4877s, Cell Signaling Technology, 1:1000), RUNX2 (sc-390351, Santa Cruz Biotechnology,1:1000) and developed with ECL (Thermo Fisher Scientific). Immunoblotting with anti-GAPDH antibody (CB1001, Emd millipore, 1:1000) was used as a loading control. Anti-OXPHOS Cocktail Kit was purchased from ThermoScientific (458099, 1:250). RNA sequencing and whole transcriptome analysis RNA-seq analysis was performed using OneStopRNAseq [67] . Specifically, FastQC [68] and MultiQC [69] were used for raw read quality control and QoRTs [70] for post-alignment quality control. Paired-end reads were aligned to mouse genome mm10, with star_2.7.5a, annotated with gencode.vM25.primary_assembly annotation [71] . Aligned exon fragments with mapping quality higher than 20 were counted toward gene expression with featureCounts_2.0.0 [72] with default settings except for the following parameters ‘-Q 20–minOverlap 1–fracOverlap 0 -p -B -C’. Differential expression (DE) analysis was performed with DESeq2_1.28.1 [73] . Within DE analysis, ’ashr’ was used to create log2 Fold Change (LFC) shrinkage for each comparison. Significant DE genes (DEGs) were filtered with the criteria FDR <0.05 and absolute log2 fold change (|LFC|) >0.585. Gene set enrichment analysis was performed with GSEA [74] . Flow cytometry analysis Bone marrow cells and splenocytes were isolated from p10 Ecsit Prx1 and Ecsit fl/fl mice. After incubation with red blood cells (RBC) lysis buffer containing NH 4 Cl, KHCO 3 , and EDTA), cells were passed through a 40 μm cell strainer, washed with FACS buffer (cold PBS (pH 7.2) containing 0.5% BSA (Fraction V) and 1 mM EDTA), and stained with mouse hematopoietic lineage antibody Cocktail (a mixture of antibodies against CD3, CD4, CD8, B220, Gr-1, CD11b and Ter119, 88–7772-72, Invitrogen, 1:100) and antibodies for cKit (12-1171-83, Invitrogen, 1:100) and Sca-1 (17-5981-82, Invitrogen, 1:100) for 30 min at 4 ˚C, washed with PBS, then 7-amino-actinomycin D (7AAD, 00-6993-50, Invitrogen, 1:1000) was added right before flow cytometry analysis to stain dead cells. Alternatively, cells were stained with Gr-1 (11-5931-85, Invitrogen, 1:100), B220 (48-0452-82, Invitrogen, 1:100), CD3ε (17-0031-82, Invitrogen, 1:100), CD11b (12-0112-82, Invitrogen, 1:100) to analyze immune cell populations. After washing three times, cells were re-suspended in cold PBS (pH 7.2) with 1 mM EDTA and analyzed with a LSRII (BD Biosciences) with the exclusion of 7AAD + cells and doublets. For flow cytometry analysis of muscle satellite cells, skeletal muscle tissues were dissected from P15 Ecsit Prx1 and Ecsit fl/fl hindlimbs and after 1 h enzymatic digestion at 37 °C, cells were stained with the following antibodies. CD45 (103103, BioLegend, 1:100), CD11b (101203, BioLegend, 1:100), Ter119 (116203, BioLegend, 1:100), Sca1 (108143, BioLegend, 1:100), integrin β-1 (102205, BioLegend, 1:100) and CXCR4 (146507, BioLegend, 1:100) for muscle-resident satellite cell staining while CD31 (102503, BioLegend, 1:100), CD45 (103103, BioLegend, 1:100), integrin-α7 (130-123-833, Miltenyi Biotec, 1:100), Sca1(108143, BioLegend, 1:100) for staining of skeletal muscle resident stem/progenitor cells. Ghost Dye (13–0865, Tonbo Biosciences, 1:100) was used to stain dead cells. For flow cytometry analysis of skeletal stem cells, P1 Ecsit Prx1 and Ecsit fl/fl limbs were dissociated by mechanical and enzymatic digestion (1mg/ml of Collagenase D (11088866001, Sigma-Aldrich), 2 mg/ml of Dispase II (4942078001, Roche), 1 mg/ml of Hyaluronidase (H3506, Sigma-Aldrich) and 10000 unit/ml of DNase I (4716728001, Roche) for 1 hour at 37 °C under gentle agitation. After blocking with purified rat anti-mouse CD16/CD32 (101302, BioLegend, 1:100) for 1 hour on ice, cells were stained with Biotin-conjugated CD45 (103103, BioLegend, 1:100), Tie2 (124005, BioLegend, 1:100) and Ter119 (116203, BioLegend, 1:100) with BV421-conjuated streptavidin (405226, BioLegend, 1:100), PE-conjugated CD51(104105, BioLegend, 1:100), BV605-conjugated Thy1.1-2 (140317, BioLegend, 1:100), APC-conjugated CD200 (123809, BioLegend, 1:100), FITC-conjugated LY51 (108305, BioLegend, 1:100) and PE/Cy7-conjugated CD105 (120409, BioLegend, 1:100) for 45 min on ice. The grating strategy of flow cytometer to analyze skeletal progenitors is described in Supplemental Fig. 3 . Alternatively, cells were isolated from P1 Ecsit ; +/+ Prx1-Cre;Rosa mT/mG , and Ecsit ; fl/fl Prx1-Cre;Rosa mT/mG limbs and stained with CD45, Tie2, and Ter119. After washing three times, cells were re-suspended in cold PBS (pH 7.2) with 1 mM EDTA and 1 µg/ml DAPI and sorted with a FACSAria II SORP cell sorter (Becton Dickinson) with exclusion of DAPI + cells and doublets. Bone fracture Bone fracture surgery was performed on 10-week-old male Osx-cre , Ecsit Osx , and Ecsit fl/fl mice. A longitudinal skin incision was made along the lateral aspect of the thigh from the stifle joint to the hip. The lateral aspect of the femur was exposed by parting the vastus lateralis muscle and the rectus femoris muscle to expose the length of the femur while preserving the femoral nerve. The middle of the femoral shaft was excised with a surgical saw. Intramedullary fixation was performed with a 25G needle penetrating from the patella furrow of the distal femur to the greater trochanter tip of the femur. Both ends of the needle were bent and then cut with a wire cutter, leaving 1 mm. Fascia was sutured using a 4/0 Vicryl suture, and then skin was closed using a 4/0 Nylon suture. Radiographs of the injured legs were performed to monitor fracture healing 2 weeks post-surgery. Ten weeks later, microCT and histology were performed for skeletal analyses. Alternatively, 6 week-old Prx1;Rosa26 mTmG mice, while still under surgical plane of anesthesia, were placed into an Einhorn Device to create a closed femoral fracture [75] , which was then confirmed by radiography. Nonunion fracture was defined as failure of bridging callus on anteroposterior and lateral fractured cortical bones by coronal and sagittal reconstruction view of microCT and radiography. Fracture unionization was defined as osseous consolidation evident on reconstruction view of microCT and radiography. AAV-mediated expression of ECSIT proteins in mice A single dose of rAAV9 vectors carrying control vector or FLAG-ECSIT constructs (2 x 10 11 GC, 50 μl) was randomly injected into P1 Ecsit fl/fl and Ecsit Prx1 neonates via the facial vein and 21 days later, skeletal and muscular phenotypes were assessed using X-ray, microCT, and histology. Alternatively, a single dose of rAAV9 vector carrying mCherry (2 x 10 11 GC, 50 μl) was injected into P1 Prx1;Rosa26 mTmG neonates via facial vein. Twenty-one days later, mCherry expression in individual tissues and the cryosectioned bone and its adjacent muscle were monitored by the IVIS-100 optical imaging and fluorescence microscopy, respectively. 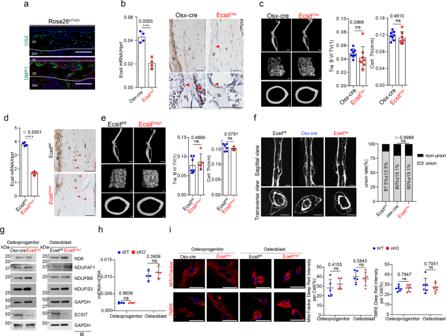Fig. 4:EcsitOsxandEcsitDmp1mice show no skeletal phenotype and intact mitochondrial function. aGFP-expressing Osterix (OSX)-, DMP1-lineage cells residing in the diaphyseal periosteum of P1Osx-EGFPandDMP1-cre;Rosa26mTmGmice, respectively, were monitored by fluorescence microscopy. m: muscle, bm: bone marrow.b,dmRNA levels ofEcsitin tibia was examined by RT-PCR (n= 4,left). Immunohistochemistry showing ECSIT expression in 2-month-oldEcsitOsx,EcsitDmp1, and littermate control femurs (right). p: periosteum, tb: trabecular bone, c: cortical bone. Red arrows indicateOsx+orDmp1+lineage osteoblasts or osteoctyes.c,eMicroCT analysis showing 3D-reconstruction images of hindlimbs, femoral trabecular and cortical bones of 2-month-oldEcsitOsx,EcsitDmp1and littermate control mice (left), and the relative quantification of trabecular bone mass (Osx-cre,EcsitOsx,n= 8;Ecsitfl/fl,n= 7;EcsitDmp1,n= 5) and cortical bone thickness (Osx-cre,n= 8;EcsitOsx,n= 7;Ecsitfl/fl,n= 6;EcsitDmp1,n= 4,right). Osx-cre limbs were used as controls forEcsitOsxmice.fMicroCT analysis showing sagittal and transverse views of fracture sites of 2-month-oldOsx-cre,EcsitOsx, andEcsitfl/flfemurs 10 weeks after the surgery, and the relative quantification of fracture union rates (n= 5).g–iOsteoprogenitors and osteoblasts were isolated fromOsx-creandEcsitOsxcalvaria andEcsitfl/flandEcsitDmp1long bones, respectively. Immunoblot analysis showing protein levels in the isolated cells. GAPDH was used as a loading control (g). A ratio of mtDNA (Ndufv1) to nDNA (18s) was assessed by RT-PCR (n= 4,h). Fluorescence microscopy shows MitoTracker- and TMRE-stained cells (i, left) and relative quantification of MitoTracker- (n= 5,i,middle) and TMRE-red signal intensity (n= 5,i,right). A two-tailed unpaired Student’st-test for comparing two groups (b,c,d,e,h,i; error bars, data represent mean ± SD) or a Fisher’s exact test (f,p> 0.9999) was applied. Data are representative of three independent experiments. Scale bars =a, 75 μm;b,d, 100 μm;c,e(left, top) 2 mm;c,e(left, middle and bottom), 100 μm;f, 1 mm;i(left), 25 μm. Mitochondrial fractionation Human bone marrow-derived stromal cells (BMSCs) were purchased from ScienCell Inc. (Cat #: 7500). Cells were resuspended in mitochondria buffer (70 mM sucrose, 1 mM EGTA, 210 mM sorbitol, 10 mM MOPS [pH 7.4]) [41] and then, the supernatant was collected after centrifugation for 10min (450g, 4 °C). For total fraction, 54 ul of the supernatant was collected after centrifugation for 10 min (550 g, 4 °C). The rest of supernatant was further centrifuged at 9500g for 10min at 4 °C and then, the supernatant was collected for the cytosol fraction. For mitochondria fraction, the pellet was resuspended in mitochondrial buffer, incubated on ice for 15 min, and centrifuged at 500 g for 10 min at 4 °C. The supernatant was further centrifuged at 9500g for 10min at 4 °C. Finally, the pellet was collected and resuspended in 54 ul mitochondria buffer as mitochondria fraction. Statistical analysis All data were presented as the mean ± SD. Sample sizes were calculated on the assumption that a 30% difference in the parameters measured would be considered biologically significant with an estimate of sigma of 10–20% of the expected mean. 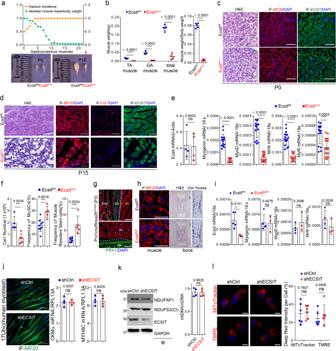Fig. 5:EcsitPrx1mice display skeletal muscle atrophy. aGraph shows the kinetics of fracture incidence and skeletal muscle weight ofEcsitPrx1andEcsitfl/flmice (n= 5,left). Representative macroscopic images of the gastrocnemius (GA) muscle at the age of P0 and P10 (right).bQuantification of skeletal muscle weight (left) and a ratio of skeletal muscle weight to body weight (right) are displayed (n= 5).c,dP0 (c) or P15 (d)EcsitPrx1andEcsitfl/fltibialis anterior (TA) muscles were stained for H&E or immunostained for MF20, COL1α1, or ECSIT.emRNA levels of myogenic genes in P10EcsitPrx1andEcsitfl/flTA muscles (n= 16).fTotal cell number (n= 5) and flow cytometry analysis showing the frequency of muscle satellite cells (MuSCs) and skeletal muscle resident stem/progenitor cells (Ecsitfl/fl,n= 9,EcsitPrx1,n= 5) in P10EcsitPrx1andEcsitfl/flGA muscles. Supplemental Fig.11demonstrates the gating strategy for this analysis.gGFP-expressing Prx1+skeletal cells in P3Prx1-cre;Rosa26mTmGGA muscle. Red: Prx1-bone marrow and muscle.h,iTibialis anterior muscles or femurs of E21EcsitMyf5andEcsitfl/flembryos were stained for H&E, Von Kossa, or immunostained for MF20 (h). mRNA levels ofEcsitand myoblast genes in the skeletal muscle (i,Ecsitfl/fl,n= 4−5;EcsitMyf5,n= 3).jHuman 17Ubic myoblasts expressing control (shCtrl) orECSITshRNA (shECSIT) were cultured under myogenic conditions. 6 days later, expression of MF20 (green) and myogenic genes was assessed (n= 4).k,lProtein levels of NDUFAF1, ECSIT and NDUFS3 (k,left) or the ratio of mtDNA (Ndufv1) to nDNA (18s,k,right) in shCtrl or shECSIT-expressing 17Ubic cells. Fluorescence microscopy shows MitoTracker- and TMRE-stained cells and relative quantification of deep red signal intensity (n= 6,l). A two-tailed unpaired Student’st-test for comparing two groups (b,e,f,i,j,k,l; error bars, data represent mean ± SD). Data are representative of three independent experiments. Scale bars =c,d, 60 μm;g, 75 μm;h, 30 μm;j, 100 μm;l, 10 μm. 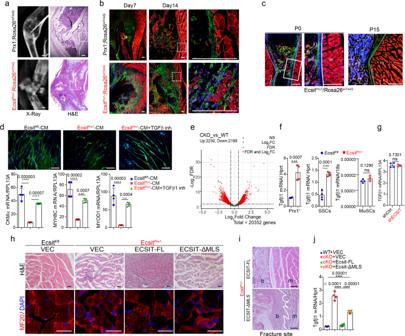Fig. 6:EcsitPrx1skeletal progenitors induce skeletal muscle degeneration. aX-radiography (left) and H&E staining (right) of P14Ecsit;Prx1Rosa26mTmGtibias with spontaneous fractures and 6-week-oldPrx1;Rosa26mTmGtibias 14 days post-fracture surgery.bFluorescence microscopy showing GFP-expressingPrx1+skeletal cells in P7 or P14Ecsit;Prx1Rosa26mTmGtibias with spontaneous fracture and 6-week-oldPrx1;Rosa26mTmGtibias 7- or 14-days post-fracture surgery. Red:Prx1-tissues.cNon-fractured sites in P0 (left) or P15 (right)Ecsit;Prx1Rosa26mTmGfemurs, demonstrating intact skeletal muscle structure. Green:Prx1+skeletal cells. Red: Prx1-bone marrow and muscle.dHuman 17Ubic myoblasts were cultured under myogenic conditions in the presence of conditioned medium (CM) harvested from the culture of FACS-sortedEcsit;Prx1Rosa26mTmG(cKO) andPrx1;Rosa26mTmG(WT) skeletal progenitors. 5 days later, expression of MF20 (green) and myogenic genes was assessed (n= 4). Alternatively, cells were treated with the TGF-β1 inhibitor SB431542.eRNA sequencing was performed on FACS-sortedEcsit;Prx1Rosa26mTmG(cKO) andPrx1;Rosa26mTmG(WT) skeletal progenitors. A volcano plot shows the gene expression for up/downregulated genes in cKO cells relative to WT cells.fmRNA levels of Tgf-β1 in FACS-sorted skeletal progenitors (left), SSCs (middle), or skeletal muscle satellite cells (MuSCs,right) (n= 4).gmRNA levels of Tgfβ1 in 17Ubic myoblast progenitors expressing control (shCtrl) orECSITshRNA (shECSIT) (n= 4).h,iAAV-treatedEcsitfl/flandEcsitPrx1TA muscles (P21) were stained for H&E (h, top) or immunostained for MF20 (h, bottom). H&E staining demonstrate intact cortical bone, periosteum, and skeletal muscle inEcsitPrx1mice expressing FLAG-tagged ECSIT-FL, not ECSIT-ΔMLS (i). White lines indicate the barrier between bone and skeletal muscle.jmRNA levels of Tgf-β1 in vector control or FLAG-ECSIT-expressing cKO and WT skeletal progenitors (n= 4). A two-tailed unpaired Student’s t-test for comparing two groups (f, g) or ordinary one-way ANOVA with Dunnett’s multiple comparisons test (d, j) (d, f, i, data represent mean ± SD). Data are representative of three independent experiments. Scale bars =a,c, 200 μm;b,d, 100 μm;h, 75 μm;i, 20 μm. Alpha and Beta were set to the standard values of .05 and 0.8, respectively. No animals or samples were excluded from analysis, and animals were randomized to treatment versus control groups, where applicable. For relevant data analysis, where relevant, we first performed the Shapiro-Wilk normality test for checking normal distributions of the groups. If normality tests passed, two-tailed, unpaired Student’s t -test were used, but if normality tests failed, Mann-Whitney tests were used for the comparisons between two groups. For the comparisons of three or four groups, we used one-way ANOVA if normality tests passed, followed by Tukey`s multiple comparison test for all pairs of groups. If normality tests failed, Kruskal–Wallis test was performed and was followed by Dunn`s multiple comparison test. For the comparison of two proportions, we performed Fisher’s exact test. The GraphPad PRISM software (v.9.4.1, La Jolla, CA) and Microsoft Office Excel 2016 were used for statistical analysis. ns, not significant; P < 0.05 was considered statistically significant. * P < 0.05; ** P < 0.01; *** P < 0.001; and **** P < 0.0001. Reporting summary Further information on research design is available in the Nature Portfolio Reporting Summary linked to this article.